The role of heterodimerization between VEGFR-1 and VEGFR-2 in the regulation of endothelial cell homeostasis VEGF-A activity is tightly regulated by ligand and receptor availability. Here we investigate the physiological function of heterodimers between VEGF receptor-1 (VEGFR-1; Flt-1) and VEGFR-2 (KDR; Flk-1) (VEGFR 1−2 ) in endothelial cells with a synthetic ligand that binds specifically to VEGFR 1−2 . The dimeric ligand comprises one VEGFR-2-specific monomer (VEGF-E) and a VEGFR-1-specific monomer (PlGF-1). Here we show that VEGFR 1−2 activation mediates VEGFR phosphorylation, endothelial cell migration, sustained in vitro tube formation and vasorelaxation via the nitric oxide pathway. VEGFR 1−2 activation does not mediate proliferation or elicit endothelial tissue factor production, confirming that these functions are controlled by VEGFR-2 homodimers. We further demonstrate that activation of VEGFR 1−2 inhibits VEGF-A-induced prostacyclin release, phosphorylation of ERK1/2 MAP kinase and mobilization of intracellular calcium from primary endothelial cells. These findings indicate that VEGFR-1 subunits modulate VEGF activity predominantly by forming heterodimer receptors with VEGFR-2 subunits and such heterodimers regulate endothelial cell homeostasis. Vascular endothelial growth factor-A (VEGF-A), a multifunctional cytokine induced by hypoxic stress [1] , initiates the assembly of endothelial cells into new blood vessels, a process known as angiogenesis, via the activation of two receptor tyrosine kinases (RTKs), VEGF receptor-1 (VEGFR-1; Flt-1) and VEGFR-2 (KDR; Flk-1) [2] . VEGF-A levels must be maintained within a narrow concentration range to ensure proper cardiovascular development and survival of the embryo [3] , [4] , [5] . The effects of VEGF-A can be deleterious if uncontrolled. Excess VEGF-A increases leakiness of blood vessels, which can cause severe oedema, loss of limb and death in animals [6] . Overexpression of VEGF-A in skeletal muscle causes hemangiomas (vascular tumours) [7] , [8] , [9] . By contrast, reduced VEGF-A activity in preeclampsia [10] , due to increased production of soluble VEGFR-1 (sFlt-1) [11] , decreases angiogenesis [12] . The varied functional activities of VEGF-A necessitate several regulatory mechanisms. In addition to sFlt-1 controlling VEGF activity [13] , membrane-bound VEGFR-1 homomeric receptor negatively regulates VEGFR-2-mediated endothelial cell proliferation [14] , [15] , [16] , [17] and tumour growth [18] . VEGFR-1 can transactivate VEGFR-2 (ref. 19 ) and an absolute requirement for VEGF receptor subtype interaction exists during the development of different blood vessels in the zebrafish embryo [20] . Heteromerization of receptor subunits is commonly observed for G-protein-coupled receptors and in RTK systems [21] , [22] . Heteromerization has been identified in the platelet-derived growth factor (PDGF) [23] and epidermal growth factor (EGF) [24] , [25] systems. Moreover, the EGF receptor subunit heterodimerizes with the PDGF-β-receptor subunit in unstimulated cells and is required for PDGF-mediated ERK1/2 phosphorylation [26] , [27] . The role of heterodimer receptors within the structurally related VEGF RTK system is ill-defined. Pre-assembled heterodimer receptors of VEGFR-2 and VEGFR-3 subunits have been isolated from primary lymphatic endothelial cells [28] , [29] and detected in situ on angiogenic sprouts [30] . Heterodimerization between VEGFR-1 and VEGFR-2 subunits (VEGFR 1−2 ) has been detected in cell-free systems [13] and in endothelial cell lines [19] , [31] , [32] , [33] . A computational model of VEGF receptor subunit dimerization concluded that a tenfold excess of one VEGF receptor subunit would result in minimal homodimerization of the less abundant receptor [34] . On the endothelial cell surface, subunits of VEGFR-1 are up to tenfold less abundant than those of VEGFR-2 (refs 35 , 36 ). This observation implies that the normal physiological state for VEGFR-1 subunits within the endothelium may be as part of heterodimers with VEGFR-2, and that VEGFR-1 in homodimer form may be relatively rare. Extensive elucidation of VEGF receptor homodimeric-specific function has been possible owing to the existence of VEGF family ligands that act selectively on the individual receptor homodimers. VEGF-B and PlGF only bind to VEGFR-1, whereas VEGF-E, a non-mammalian viral protein, is a selective agonist for VEGFR-2. The native forms of VEGF-C and VEGF-D are VEGFR-3-specific. In vivo , VEGFR 1−2 is activated by VEGF-A and the VEGF-A:PlGF-1 heterodimer, but these ligands also simultaneously activate VEGF homodimeric receptors. Currently, no natural ligands are known that exclusively activate VEGFR 1−2 without activating VEGFR-1 homodimers. Therefore, dissection of VEGFR 1−2 heterodimer-specific function has been challenging. Receptor subunit knockdown and use of cell lines expressing specific receptors indicate that prostacyclin release [33] and biphasic calcium induction [32] is likely to be the result of VEGFR 1−2 activation. To investigate the function of VEGFR 1−2 in endothelial cells, we have generated a novel, VEGFR 1−2 -specific ligand (VEGF-E:PlGF-1), comprising one monomer of VEGFR-2-specific ligand (VEGF-E) and one monomer of PlGF-1, a specific ligand for VEGFR-1. We show that the heterodimer mediates responses previously shown to involve VEGFR-1 homodimers and negatively regulates some VEGFR-2-mediated functions. Thus, VEGFR-1 subunits seem to regulate VEGF activity predominantly by forming heterodimer receptors with VEGFR-2 subunits to maintain endothelial cell homeostasis. Receptor nomenclature in this manuscript follows the recommendations from Ferre and co-workers [37] . A 'receptor' is defined as the minimal functional, signal-transducing unit and, for RTKs, this normally comprises two subunits. Therefore, a 'homomer/homodimer receptor' is the minimal functional unit comprised of two or more of the same subunits that are not functional on their own. VEGFR-1 and VEGFR-2 form heterodimers in endothelial cells Heterodimerization between VEGFR-1 and VEGFR-2 subunits in preassembled complexes has been identified in cell-free systems [13] and in porcine [32] , bovine [33] and murine [19] endothelial cell lines. We confirmed VEGF receptor subunit heterodimerization in porcine aortic endothelial cells (PAEC) overexpressing human VEGFR-1 and VEGFR-2 (PAER-1:R-2), by immunoprecipitation ( Fig. 1a ; Supplementary Fig. S1 for full-length blot). To date, evidence for VEGFR 1−2 heterodimers in primary human endothelial cells has been lacking. Using the immunoprecipitation procedure optimized with the PAEC we successfully demonstrated that VEGFR-1 and VEGFR-2 subunits do heterodimerize in an immortalized human endothelial cell line (HMEC-1) and in primary human endothelial cells (HUVEC) ( Fig. 1b ). In addition, VEGFR-2 could be detected in VEGFR-1 immunoprecipitates ( Fig. 1c ) and co-localization of the two receptors in HUVEC was shown by confocal microscopy ( Fig. 1d ). Enzyme-linked immunosorbent assay (ELISA) further confirmed the presence of preassembled VEGFR 1−2 heterodimers in human endothelial cells ( Fig. 1e ) and in the mouse liver, lung and kidney ( Fig. 1f ). 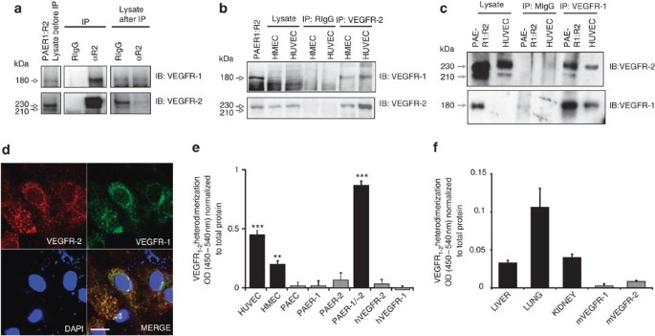Figure 1: VEGFR1−2heterodimerization in human endothelial cells. Lysates of (a) PAER-1 cells, and (b) HMEC-1 and HUVEC cells were immunoprecipitated with anti-VEGFR-2 or rabbit IgG and Western-blotted for VEGFR-1 or VEGFR-2. (c) PAER-1:R-2 cells and HUVEC were immunoprecipitated with anti-VEGFR-1 or mouse IgG and western-blotted for VEGFR-1 or VEGFR-2. (d) Confocal microscopy showing a representative image of VEGFR-1 co-localized with VEGFR-2, in HUVEC. Scale bar, 20 μm. (e) VEGFR1−2heterodimerization was assayed in cell lysates by ELISA. (f) VEGFR1−2heterodimerization was assayed in lysates from mouse organs. Results are expressed as mean (+s.e.m.) of at least three independent experiments. **P<0.01 versus PAER-2, ***P<0.001 versus PAER-2. Figure 1: VEGFR 1−2 heterodimerization in human endothelial cells. Lysates of ( a ) PAER-1 cells, and ( b ) HMEC-1 and HUVEC cells were immunoprecipitated with anti-VEGFR-2 or rabbit IgG and Western-blotted for VEGFR-1 or VEGFR-2. ( c ) PAER-1:R-2 cells and HUVEC were immunoprecipitated with anti-VEGFR-1 or mouse IgG and western-blotted for VEGFR-1 or VEGFR-2. ( d ) Confocal microscopy showing a representative image of VEGFR-1 co-localized with VEGFR-2, in HUVEC. Scale bar, 20 μm. ( e ) VEGFR 1−2 heterodimerization was assayed in cell lysates by ELISA. ( f ) VEGFR 1−2 heterodimerization was assayed in lysates from mouse organs. Results are expressed as mean (+s.e.m.) of at least three independent experiments. ** P <0.01 versus PAER-2, *** P <0.001 versus PAER-2. Full size image Production and purification of a VEGFR 1 − 2 -specific ligand To characterize the function of the VEGFR 1−2 heterodimer, we engineered a dimeric ligand that exclusively binds to this receptor. The ligand was produced using the insect cell-baculovirus system and comprises one monomer of VEGFR-2-specific VEGF-E and one monomer of His-Tagged, VEGFR-1-specific, human PlGF-1. VEGF-E is a viral protein, identified in a number of strains of the orf virus, which has the ability to specifically bind to and activate VEGFR-2 (ref. 38 ). The VEGF-E isoform used, in this study, was isolated from the D1701 strain [39] and was engineered to contain the VEGF-A-heparin-binding domain [40] . This protein binds to both heparin and neuropilin-1 like VEGF-A [40] . Purification of the novel recombinant heterodimeric ligand was achieved by sequential application of the medium to Ni-NTA and Heparin-Sepharose columns. The antibodies against VEGF-E and PlGF did not cross-react and the two proteins migrated differently (PlGF as two bands at 21 kDa and 22 kDa and VEGF-E at 23 kDa; Fig. 2a ). Both proteins were expressed after simultaneous infection of the same cells with both viruses ( Fig. 2b ) and ELISA demonstrated heterodimerization of VEGF-E subunits with those of PlGF-1 after the infection ( Fig. 2c ). Samples of the purified proteins of PlGF-1, VEGF-E:PlGF-1 and VEGF-E were run adjacently on SDS–PAGE under reduced and non-reduced conditions to ascertain protein size and reactivity with the PlGF and VEGF-E antibodies. Silver staining showed that the heterodimer preparation was ~95% pure ( Fig. 2d ). Under non-reducing conditions, the novel ligand migrated to an intermediate distance between PlGF-1 and VEGF-E at 43 kDa ( Fig. 2d ) and it reacted with antibodies against PlGF-1 and VEGF-E ( Fig. 2d ), confirming the purification of the heterodimeric ligand. To assess the binding capacity of the novel ligand to endothelial cells, PAER-1:R-2 were incubated with VEGF-E:PlGF-1 and binding detected using an anti-His-Tag antibody by fluorescence-activated cell sorting (FACS). Endothelial cells express PlGF, so the anti-His-Tag antibody was used to distinguish endogenous cell surface PlGF from the novel ligand. The presence of VEGF-E:PlGF-1 was demonstrated on the cell surface of PAER-1:R-2 ( Fig. 2e , bottom right), but not on PAEC, which lack VEGF receptors ( Fig. 2e top left), PAER-1 ( Fig. 2e , top right) or PAER-2 ( Fig. 2e , bottom left), demonstrating that VEGF-E:PlGF-1 specifically binds to the VEGFR 1−2 heterodimer receptor. 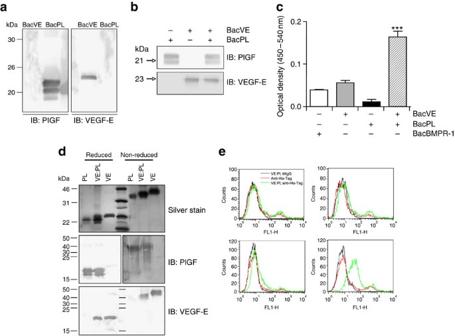Figure 2: Production and purification of VEGF-E:PlGF-1. (a) Western blotting of supernatants taken from Sf 21 insect cells infected for three days with baculoviruses encoding either PlGF-1 or VEGF-E, confirmed absence of cross-reactivity between the antibodies. One-half of the membrane was immunoblotted with anti-PlGF (172) and the other with anti-VEGF-E antibodies. (b) Simultaneous infection of Sf 21 cells with both baculoviruses led to expression of both VEGF-E and PlGF-1. (c) Plates were coated with anti-His-Tag antibody and VEGF-E:PlGF-1 heterodimers detected in supernatants from Sf 21 insect cells after single and dual infections with baculoviruses encoding PlGF-1 and VEGF-E using anti-VEGF-E antibodies. Supernatant from Bac-BMPR-1 (irrelevant protein)-infected cells was used as a negative control. (d) Samples of recombinant PlGF-1, VEGF-E:PlGF-1 or heparin-binding VEGF-E (100 ng per lane) were subjected to SDS–PAGE and gels either stained with silver stain for total protein, or proteins were transferred to membranes for western blotting with anti-VEGF-E or anti-PlGF-1, under reducing or non-reducing conditions. ***P<0.001 versus Bac-VEGF-E, alone. (e) PAEC (top left), PAER-1 (top right), PAER-2 (bottom left) and PAER-1:R-2 (bottom right) were incubated with VEGF-E:PlGF-1 (100 ng per 2.5×106cells) and binding detected with anti-His-Tag antibody by FACS. Results are expressed as mean (+s.e.m.) of at least three independent experiments. Figure 2: Production and purification of VEGF-E:PlGF-1. ( a ) Western blotting of supernatants taken from Sf 21 insect cells infected for three days with baculoviruses encoding either PlGF-1 or VEGF-E, confirmed absence of cross-reactivity between the antibodies. One-half of the membrane was immunoblotted with anti-PlGF (172) and the other with anti-VEGF-E antibodies. ( b ) Simultaneous infection of Sf 21 cells with both baculoviruses led to expression of both VEGF-E and PlGF-1. ( c ) Plates were coated with anti-His-Tag antibody and VEGF-E:PlGF-1 heterodimers detected in supernatants from Sf 21 insect cells after single and dual infections with baculoviruses encoding PlGF-1 and VEGF-E using anti-VEGF-E antibodies. Supernatant from Bac-BMPR-1 (irrelevant protein)-infected cells was used as a negative control. ( d ) Samples of recombinant PlGF-1, VEGF-E:PlGF-1 or heparin-binding VEGF-E (100 ng per lane) were subjected to SDS–PAGE and gels either stained with silver stain for total protein, or proteins were transferred to membranes for western blotting with anti-VEGF-E or anti-PlGF-1, under reducing or non-reducing conditions. *** P <0.001 versus Bac-VEGF-E, alone. ( e ) PAEC (top left), PAER-1 (top right), PAER-2 (bottom left) and PAER-1:R-2 (bottom right) were incubated with VEGF-E:PlGF-1 (100 ng per 2.5×10 6 cells) and binding detected with anti-His-Tag antibody by FACS. Results are expressed as mean (+s.e.m.) of at least three independent experiments. Full size image VEGF-E:PlGF-1 induces VEGFR-2 and ERK1/2 phosphorylation To assess whether the VEGF-E:PlGF-1 ligand increases VEGFR 1−2 heterodimers to levels above those already preassembled, lysates of HUVEC stimulated with VEGF-E:PlGF-1 were immunoprecipitated with anti-VEGFR-2 and immunoblotted with anti-VEGFR-1 ( Fig. 3a ), or subjected to the human VEGFR 1−2 ELISA ( Fig. 3b ). No increase in VEGFR 1−2 was detected after addition of VEGF-E:PlGF-1 in either assay. It is possible that our assays were not sensitive enough to detect an increase in heterodimerization. However, these findings support the computational model of VEGF receptor dimerization, which states that when an excess of one receptor subunit is present, most of the less abundant receptor subunit will be present as preassembled heterodimers with it [34] . 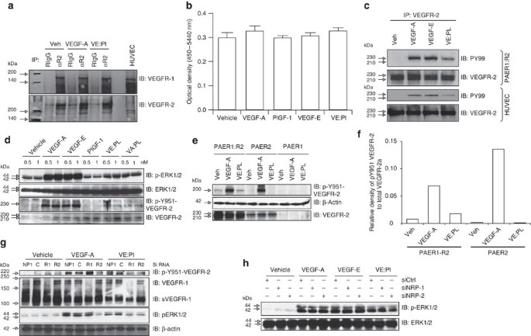Figure 3: Effect of VEGF-E:PlGF-1 on receptor heterodimerization and phosphorylation of VEGFR-2 and ERK1/2. (a) HUVEC were stimulated with vehicle, VEGF-A or VEGF-E:PlGF-1 for 15 min. Cell lysates were immunoprecipitated with anti-VEGFR-2 or rabbit IgG control antibodies and western-blotted for VEGFR-1. In parallel ,a western blot was performed to control for VEGFR-2 concentration in the immunoprecipitates. (b) HUVEC were stimulated with VEGF-A, PlGF-1, VEGF-E and VEGF-E:PlGF-1 for 15 min. VEGFR1−2heterodimerization was assessed by ELISA. (c) PAER-1:R-2 cells and HUVEC were rested for 24 h and 12 h, respectively and stimulated for 15 min with, VEGF-A, VEGF-E or VEGF-E:PlGF-1. Lysates were immunoprecipitated with anti-VEGFR-2 and western-blotted for phospho-tyrosine (PY99), then stripped and reprobed with anti-VEGFR-2. (d) HUVEC were incubated with growth factors for 10 min and cell lysates western-blotted for phosphorylated ERK1/2 (p-ERK1/2), ERK1/2, phosphorylated VEGFR-2 tyrosine 951 (p-Y951-VEGFR-2) and VEGFR-2. (e) PAER-1, PAER-2 and PAER-1:R-2 were incubated with equimolar concentrations of VEGF-A or VEGF-E:PlGF for 5 min. The cell lysates were probed for phosphorylated VEGFR-2 tyrosine 951 (p-Y951-VEGFR-2), VEGFR-2 and, β-actin. (f) Densitometric analysis of VEGFR-2 phosphorylation shown ine. (g) VEGFR-1, VEGFR-2 and neuropilin-1 were knocked down in HUVEC by transfection with siRNA using an AMAXA nucleofector. Cells were then incubated with VEGF-A, VEGF-A:PlGF for 5 min and lysates probed for p-Y951-VEGFR-2, VEGFR-1 p-ERK1/2 and β-actin. (h) Neuropilin-1 and neuropilin-2 were knocked down in HUVEC using siRNA. Cells were then incubated with VEGF-A, VEGF-E VEGF-A:PlGF for 15 min. Lysates were probed for phosphorylated p-ERK1/2 and ERK1/2. Results are expressed as mean (+s.e.m.) of at least three independent experiments. Figure 3: Effect of VEGF-E:PlGF-1 on receptor heterodimerization and phosphorylation of VEGFR-2 and ERK1/2. ( a ) HUVEC were stimulated with vehicle, VEGF-A or VEGF-E:PlGF-1 for 15 min. Cell lysates were immunoprecipitated with anti-VEGFR-2 or rabbit IgG control antibodies and western-blotted for VEGFR-1. In parallel ,a western blot was performed to control for VEGFR-2 concentration in the immunoprecipitates. ( b ) HUVEC were stimulated with VEGF-A, PlGF-1, VEGF-E and VEGF-E:PlGF-1 for 15 min. VEGFR 1−2 heterodimerization was assessed by ELISA. ( c ) PAER-1:R-2 cells and HUVEC were rested for 24 h and 12 h, respectively and stimulated for 15 min with, VEGF-A, VEGF-E or VEGF-E:PlGF-1. Lysates were immunoprecipitated with anti-VEGFR-2 and western-blotted for phospho-tyrosine (PY99), then stripped and reprobed with anti-VEGFR-2. ( d ) HUVEC were incubated with growth factors for 10 min and cell lysates western-blotted for phosphorylated ERK1/2 (p-ERK1/2), ERK1/2, phosphorylated VEGFR-2 tyrosine 951 (p-Y951-VEGFR-2) and VEGFR-2. ( e ) PAER-1, PAER-2 and PAER-1:R-2 were incubated with equimolar concentrations of VEGF-A or VEGF-E:PlGF for 5 min. The cell lysates were probed for phosphorylated VEGFR-2 tyrosine 951 (p-Y951-VEGFR-2), VEGFR-2 and, β-actin. ( f ) Densitometric analysis of VEGFR-2 phosphorylation shown in e . ( g ) VEGFR-1, VEGFR-2 and neuropilin-1 were knocked down in HUVEC by transfection with siRNA using an AMAXA nucleofector. Cells were then incubated with VEGF-A, VEGF-A:PlGF for 5 min and lysates probed for p-Y951-VEGFR-2, VEGFR-1 p-ERK1/2 and β-actin. ( h ) Neuropilin-1 and neuropilin-2 were knocked down in HUVEC using siRNA. Cells were then incubated with VEGF-A, VEGF-E VEGF-A:PlGF for 15 min. Lysates were probed for phosphorylated p-ERK1/2 and ERK1/2. Results are expressed as mean (+s.e.m.) of at least three independent experiments. Full size image To assess whether the novel ligand could induce receptor phosphorylation, PAER-1:R-2 and HUVEC were stimulated with VEGF-A, VEGF-E and VEGF-E:PlGF-1. Lysates were immunoprecipitated with anti-VEGFR-2, or anti-VEGFR-1 and immunoblotted for phosphorylated tyrosine residues. Tyrosine phosphorylation of VEGFR-2 was detected after stimulation with VEGF-A, VEGF-E and VEGF-E:PlGF-1 in PAER-1:R-2 and in HUVEC ( Fig. 3c,d ). Stimulation of HUVEC with equimolar concentrations of VEGF-A and VEGF-E induced strong phosphorylation of ERK1/2 MAPK, whereas VEGF-E:PlGF-1 only induced a weak ERK1/2 phosphorylation ( Fig. 3d ). VEGF-E:PlGF-1 could not induce VEGFR-2 phosphorylation in PAER-2 cells ( Fig. 3e ) confirming the absence of contaminating VEGF-E homodimers in the ligand preparation and indicating that the presence of both receptors is required for the signalling activity of VEGF-E:PlGF-1. The PAER-1:R-2 cell line was produced by stably transfecting PAER-2 with human VEGFR-1, thus PAER-2 are the parent cells of PAER-1:R-2 cells. However, when equal protein concentrations of lysates were probed for total VEGFR-2, VEGFR-2 levels were found to be lower in PAER-2 cells compared with PAER-1:R-2 cells ( Fig. 3e ). The decreased expression of VEGFR-2 in PAER-2 cells was confirmed in different batches of the cells by western blotting ( Supplementary Fig. S2A ) and ELISA for human VEGFR-2 ( Supplementary Fig. S2B ). These interesting findings suggest that VEGFR-1 stabilizes VEGFR-2 in the cell. It is likely to be a structural feature of VEGFR-1 that stabilizes VEGFR-2 as mutation of VEGFR-1 tyrosine 1213, which is critical for VEGFR-1 function, did not affect VEGFR-2 levels in PAER-1:R-2 cells ( Supplementary Fig. S2B ). In addition, mutation of this tyrosine had no effect on the level of VEGFR-1 ( Supplementary Fig. S2C) or heterodimerization within PAEC containing both receptors ( Supplementary Fig. S2D ). In addition, densitometric analysis indicated that phosphorylation of VEGFR-2 was greater in cells lacking VEGFR-1 ( Fig. 3f ). Short interfering RNA (siRNA)-mediated knockdown of VEGFR-1 in HUVEC (knockdown verified by western blotting; Fig. 3g ) caused a big increase in VEGFR-2 phosphorylation ( Fig. 3g ). Interestingly, ERK1/2 MAPK phosphorylation was comparable to siRNA control-transfected samples, but this was likely due to the stimulation time point being too short. Knockdown of either VEGFR-1 or VEGFR-2 ( Supplementary Fig. S3A for ELISA verifying VEGFR-2 knockdown) inhibited the ability of VEGF-E:PlGF-1 to induce VEGFR-2 and ERK1/2 phosphorylation ( Fig. 3g ). Showing changes in the phosphorylation status of VEGFR-1 is particularly difficult [41] , [42] . We attempted to ascertain VEGFR-1 phosphorylation status following VEGF-A or PlGF-1 or VEGF-E:PlGF-1 stimulation of PAER-1:R-2. No increase in VEGFR-1 tyrosine phosphorylation was detected by either immunoprecipitation or VEGFR-1 phospho-tyrosine ELISA. Neuropilins have no role in VEGF-E:PlGF-1-induced signalling The heparin-binding domain of VEGF confers the ability to interact with two co-receptors; neuropilin-1 and -2 (NRP-1 and NRP-2). Although, VEGF cannot induce neuropilin phosphorylation or signalling, neuropilins have been shown to associate with the VEGF receptors [43] . This is reported to augment the functional response to VEGF in endothelial cells [43] . To ascertain whether neuropilins have any role in heterodimer receptor function, we used siRNA to knockdown neuropilin-1 and neuropilin-2 in HUVEC and then stimulated with the ligand. Neuropilin-1 knockdown had no effect on VEGFR-2 phosphorylation after VEGF-A or VEGF-E:PLGF-1 administration ( Fig. 3g ) and knockdown of neuropilin-1 or neuropilin-2 had no effect on ERK1/2 phosphorylation ( Fig. 3h ). This suggests neuropilins are not having a major role for these signalling functions. (Verification of neuropilin-1 and neuropilin-2 knockdown can be seen in Supplementary Fig. 3c,d ). Whether neuropilins are involved at a functional level warrants further enquiry. Ligand and receptor dynamics To assess cellular binding and trafficking of VEGF-E:PlGF-1, HUVEC treated with the ligand for 2.5–120 min. were stained with the anti-VEGF-E antibody without permeabilization. Confocal microscopy analysis demonstrated that VEGF-E:PlGF-1 bound to the cell but was undetectable by 30–60 min ( Fig. 4a ). Following 15 min of stimulation, VEGF-E:PlGF-1 was detected within the cell indicating internalization of the ligand ( Fig. 4b ). Interestingly, the staining pattern was strikingly different between cells stimulated with VEGF-E and those stimulated with VEGF-E:PlGF-1. VEGF-E seemed to be predominantly located in the nucleus, whereas VEGF-E:PlGF-1 was diffusely distributed throughout the intracellular compartment ( Fig. 4b ). 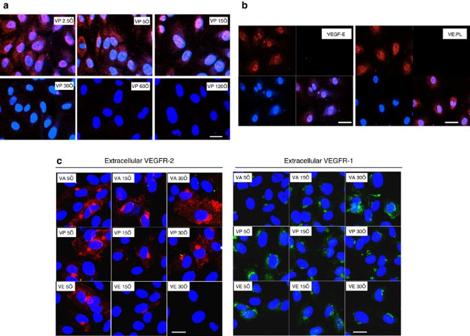Figure 4: Distribution of ligands and receptors in response to VEGF-E:PlGF-1. (a) Time course of VEGF-E:PlGF-1 stimulation of HUVEC, showing the presence of VEGF-E:PlGF-1 on the cell surface, detected with anti-VEGF-E using confocal microscopy. Scale bar, 20 μm. (b) Intracellular localization of VEGFR-2 in HUVEC after stimulation with VEGF-E and VEGF-E:PlGF-1 for 15 min. Scale bar, 40 μm. (c) Time course showing a comparison of VEGFR-1 and VEGFR-2 distribution on the cell surface post-stimulation with VEGF-A, VEGF-E and VEGF-E:PlGF-1. Scale bar, 20 μm. Figure 4: Distribution of ligands and receptors in response to VEGF-E:PlGF-1. ( a ) Time course of VEGF-E:PlGF-1 stimulation of HUVEC, showing the presence of VEGF-E:PlGF-1 on the cell surface, detected with anti-VEGF-E using confocal microscopy. Scale bar, 20 μm. ( b ) Intracellular localization of VEGFR-2 in HUVEC after stimulation with VEGF-E and VEGF-E:PlGF-1 for 15 min. Scale bar, 40 μm. ( c ) Time course showing a comparison of VEGFR-1 and VEGFR-2 distribution on the cell surface post-stimulation with VEGF-A, VEGF-E and VEGF-E:PlGF-1. Scale bar, 20 μm. Full size image HUVEC were treated with VEGF-A, VEGF-E and VEGF-E:PlGF-1, and the distribution of the receptors evaluated using antibodies raised against the amino-termini of VEGFR-1 and VEGFR-2. VEGFR-1 expression remained stable at the cell surface throughout the stimulation period ( Fig. 4c ). By contrast, VEGFR-2 rapidly disappeared from the cell surface after stimulation with VEGF-E ( Fig. 4c ), whereas VEGFR-2 levels following stimulation with VEGF-A and VEGF-E:PlGF-1, which bind to VEGFR 1−2 remained at the cell surface ( Fig. 4c ), further supporting to our earlier findings that the activation of VEGFR-1 can stabilize VEGFR-2 levels. Functional consequences of VEGFR 1 − 2 activation Existing research using ligands specific for VEGFR-1 or VEGFR-2 homomeric receptors and cell lines expressing only a single receptor subunit type demonstrates that VEGF-A-mediated endothelial cell migration [16] , [42] , and induction of VEGFR-1 promoter activity and tissue factor release [44] , are VEGFR-2-mediated functions. However, the limitation of these tools is that they cannot fully delineate the contribution of VEGFR 1−2 to these functions. Use of VEGF-E:PlGF-1 in a modified Boyden chamber assay demonstrated that VEGFR 1−2 activation is involved in the migration of human primary endothelial cells ( Fig. 5a ). VEGF-E:PlGF-1 could not induce migration of PAER-2 ( Fig. 5b ) confirming the absence of VEGF-E contamination in the purified fraction. VEGF-E:PlGF-1 induced activity of a VEGFR-1 promoter luciferase reporter construct in cells containing both VEGFR-1 and VEGFR-2 subunits, but not in cells only expressing VEGFR-2 ( Fig. 5c ). VEGF-E:PlGF-1 also caused release of sVEGFR-1 from HUVEC ( Fig. 5d ), demonstrating the VEGFR 1−2 signal results in a regulatory function. 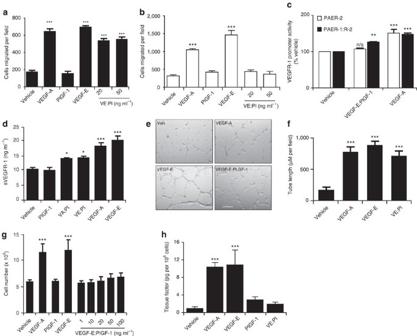Figure 5: Effect of VEGF-E:PlGF-1 on endothelial cell function. Migration of (a), HUVEC and (b) PAER-2 cells in response to VEGF-A, PlGF-1, VEGF-E and VEGF-E:PlGF-1 (VE:Pl) was assessed using a modified Boyden chamber assay. ***P<0.001 versus control. (c) PAER-2 and PAER-1:R-2 cells were transfected with a VEGFR-1 promoter reporter construct and incubated with VEGF-E:PlGF-1 or VEGF-A for 30 h and promoter activity determined by dual luciferase assay. **P<0.01 versus vehicle. (d) HUVEC were incubated with growth factors for 24 h and sFlt-1 (sVEGFR-1) release into the media was assayed by ELISA. (e) HUVEC were seeded on growth factor-reduced Matrigel and allowed to attach for 4 h. Cells were incubated with Vehicle (top left), VEGF-A (top right), VEGF-E (bottom left) and VEGF-E:PlGF-1 (bottom right) and development of tube-like structures assessed every 2 h. Scale bar, 150 μm. (f) After 18 h, tube length per field quantified in 10 random 10 power fields. ***P<0.001 versus vehicle. (g) HUVEC were rested overnight before treatment with; vehicle, VEGF-A, PlGF-1, hbVEGF-E and VEGF-E:PlGF-1. After 96 h, an MTT assay was performed and absorbance equated to cell number. ***P<0.001 versus control. (h) Confluent HUVEC were rested overnight and stimulated with vehicle VEGF-A, PlGF-1, VEGF-E and VEGF-E:PlGF-1 (VE:Pl) for 6 h and a coagulation assay used to determine tissue factor production. ***P<0.001 versus vehicle. Results are expressed as mean (+s.e.m.) of at least three independent experiments. Figure 5: Effect of VEGF-E:PlGF-1 on endothelial cell function. Migration of ( a ), HUVEC and ( b ) PAER-2 cells in response to VEGF-A, PlGF-1, VEGF-E and VEGF-E:PlGF-1 (VE:Pl) was assessed using a modified Boyden chamber assay. *** P <0.001 versus control. ( c ) PAER-2 and PAER-1:R-2 cells were transfected with a VEGFR-1 promoter reporter construct and incubated with VEGF-E:PlGF-1 or VEGF-A for 30 h and promoter activity determined by dual luciferase assay. ** P <0.01 versus vehicle. ( d ) HUVEC were incubated with growth factors for 24 h and sFlt-1 (sVEGFR-1) release into the media was assayed by ELISA. ( e ) HUVEC were seeded on growth factor-reduced Matrigel and allowed to attach for 4 h. Cells were incubated with Vehicle (top left), VEGF-A (top right), VEGF-E (bottom left) and VEGF-E:PlGF-1 (bottom right) and development of tube-like structures assessed every 2 h. Scale bar, 150 μm. ( f ) After 18 h, tube length per field quantified in 10 random 10 power fields. *** P <0.001 versus vehicle. ( g ) HUVEC were rested overnight before treatment with; vehicle, VEGF-A, PlGF-1, hbVEGF-E and VEGF-E:PlGF-1. After 96 h, an MTT assay was performed and absorbance equated to cell number. *** P <0.001 versus control. ( h ) Confluent HUVEC were rested overnight and stimulated with vehicle VEGF-A, PlGF-1, VEGF-E and VEGF-E:PlGF-1 (VE:Pl) for 6 h and a coagulation assay used to determine tissue factor production. *** P <0.001 versus vehicle. Results are expressed as mean (+s.e.m.) of at least three independent experiments. Full size image Capillary-like tube formation on growth factor-reduced Matrigel requires endothelial cell differentiation and survival. HUVEC were seeded on matrigel and stimulated with VEGF ligands for 18 h. VEGF-E:PlGF-1 significantly induced in vitro tube formation to similar levels as that observed with VEGF-A and VEGF-E ( Fig. 5e,f ) suggesting that VEGFR 1−2 heterodimer signalling is important for angiogenesis. VEGF-A induces endothelial cell proliferation as a direct result of VEGFR-2-mediated ERK1/2 MAPK phosphorylation [45] . Stimulation of HUVEC with VEGF-A and VEGF-E resulted in a significant increase in proliferation ( Fig. 5g ) consistent with the observed strong ERK1/2 phosphorylation ( Fig. 3d,g ). By contrast, VEGF-E:PlGF-1 induced only weak ERK1/2 phosphorylation ( Fig. 3d,g ) and did not induce cell proliferation ( Fig. 5g ), indicating that VEGFR-2 homodimer activation is required for the VEGF-mediated proliferative response. Tissue factor expression and subsequent coagulation has been attributed to VEGFR-2 (ref. 44 ). VEGF-E:PlGF-1 did not induce tissue factor expression, confirming the VEGFR-2 specificity of this response ( Fig. 5h ). VEGF-E:PlGF-1 modulates vessel reactivity An important function of VEGF-A is the regulation of vascular tone. After precontraction, VEGF-E:PlGF-1, PlGF-1 and VEGF-A caused vasorelaxation of arterial tissue ( Fig. 6a ). Relaxation could be abolished by co-incubation with L -NAME ( Fig. 6b–d ), confirming the role of endothelial-derived nitric oxide (NO) in vascular relaxation. Interestingly, activation of the VEGFR-2 homodimer by VEGF-E did not significantly alter vascular tone within the same concentration range as the other VEGF ligands (≤1 nM; Fig. 6a ); providing evidence, for the first time, that VEGF-A-induced vasorelaxation may depend on the VEGFR-1 homodimer and/or the VEGFR 1−2 heterodimer and that the VEGFR-1 homodimer is not involved. 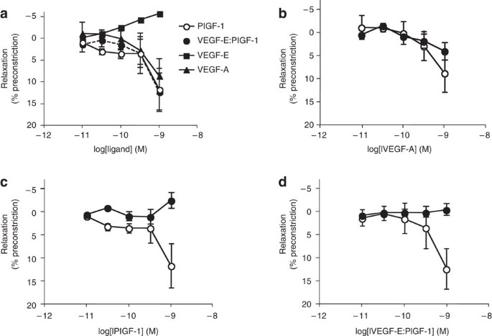Figure 6: Vasorelaxation induced by VEGF ligands in isolated rat aorta. (a) VEGF-E:PlGF-1, PlGF-1 and VEGF-A, but not VEGF-E, cause vasorelaxation. The relaxation to (b) VEGF-A, (c) PlGF-1 and (d) VEGF-E:PlGF-1 is inhibited by Nω-Nitro-L-arginine methyl ester (L-NAME; 200 μM) supporting a role for NO in this response. Control (open circles),L-NAME (black circles). Vessels are precontracted with EC80phenylephrine and relaxation expressed as a percentage of the precontraction. Data points are means s.e.m. Results are expressed as mean (+s.e.m.) of at least three independent experiments. Figure 6: Vasorelaxation induced by VEGF ligands in isolated rat aorta. ( a ) VEGF-E:PlGF-1, PlGF-1 and VEGF-A, but not VEGF-E, cause vasorelaxation. The relaxation to ( b ) VEGF-A, ( c ) PlGF-1 and ( d ) VEGF-E:PlGF-1 is inhibited by N ω -Nitro- L -arginine methyl ester ( L -NAME; 200 μM) supporting a role for NO in this response. Control (open circles), L -NAME (black circles). Vessels are precontracted with EC 80 phenylephrine and relaxation expressed as a percentage of the precontraction. Data points are means s.e.m. Results are expressed as mean (+s.e.m.) of at least three independent experiments. Full size image It is well established that VEGF-A is important for the release of the vasodilator NO, and that NO is crucial for VEGF-A-mediated angiogenesis [14] , [16] , [42] , [46] , [47] . To ascertain whether VEGFR 1−2 has a direct role in NO release, supernatants from VEGF-E:PlGF-1 stimulated HUVEC were assayed for NO content, using a Sievers NOA 280 chemiluminescence analyser. VEGF-E:PlGF-1 induced NO release from HUVEC in a concentration-dependent manner ( Fig. 7a ) and stimulated eNOS activation as indicated by an increase in phosphorylation of eNOS at serine-1177 ( Fig, 7b ). 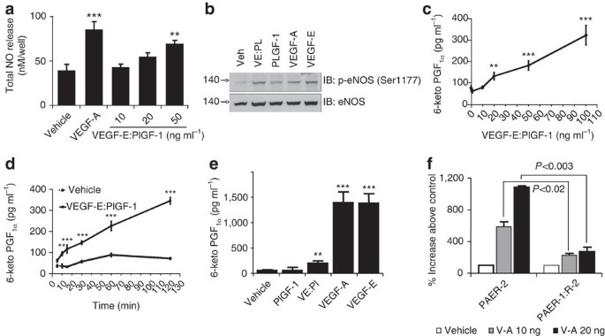Figure 7: VEGF-E:PlGF-1 causes NO and prostacyclin release. (a) Human umbilical vein endothelial cells (HUVEC) were rested overnight before stimulation with vehicle, VEGF-A or VEGF-E:PlGF-1 for 1 h and supernatant analysed for NO content using a Sievers NOA 280 chemiluminescence analyzer. (b) HUVEC lysates were then subjected to SDS–PAGE and western-blotted with anti phospho-eNOS serine 1177 (p-eNOS (serine 1177)) and eNOS. (c) HUVEC were incubated with increasing concentrations of VEGF-E:PlGF-1 or (d), with VEGF-E:PlGF-1 (50 ng ml−1) for increasing time periods and 6-keto PGF1αwas assessed in the supernatants by ELISA. **P<0.01 versus vehicle. ***P<0.001 versus vehicle. (e) Treatment with vehicle, VEGF-A, PlGF-1, VEGF-E and VEGF-E:PlGF-1 (VE:Pl). After 30 min, supernatant was collected and assayed for 6-keto-PGF1αby ELISA. **P<0.01 or ***P<0.0001 versus vehicle. (f) PAER-2 and PAER-1:R-2 were rested for 24 h before incubation with VEGF-A for 30 min. Supernatant was collected and 6-keto PGF1αwas assessed by ELISA. Results are expressed as mean (+s.e.m.) of at least three independent experiments. Figure 7: VEGF-E:PlGF-1 causes NO and prostacyclin release. ( a ) Human umbilical vein endothelial cells (HUVEC) were rested overnight before stimulation with vehicle, VEGF-A or VEGF-E:PlGF-1 for 1 h and supernatant analysed for NO content using a Sievers NOA 280 chemiluminescence analyzer. ( b ) HUVEC lysates were then subjected to SDS–PAGE and western-blotted with anti phospho-eNOS serine 1177 (p-eNOS (serine 1177)) and eNOS. ( c ) HUVEC were incubated with increasing concentrations of VEGF-E:PlGF-1 or ( d ), with VEGF-E:PlGF-1 (50 ng ml −1 ) for increasing time periods and 6-keto PGF 1α was assessed in the supernatants by ELISA. ** P <0.01 versus vehicle. *** P <0.001 versus vehicle. ( e ) Treatment with vehicle, VEGF-A, PlGF-1, VEGF-E and VEGF-E:PlGF-1 (VE:Pl). After 30 min, supernatant was collected and assayed for 6-keto-PGF 1α by ELISA. ** P <0.01 or *** P <0.0001 versus vehicle. ( f ) PAER-2 and PAER-1:R-2 were rested for 24 h before incubation with VEGF-A for 30 min. Supernatant was collected and 6-keto PGF 1α was assessed by ELISA. Results are expressed as mean (+s.e.m.) of at least three independent experiments. Full size image The VEGF-mediated release of prostacyclin from endothelial cells was previously attributed to VEGFR 1−2 activation [33] . Consistent with this report, stimulation of HUVEC with VEGF-E:PlGF-1 induced a time-dependent and concentration-dependent increase in prostacyclin release as measured by the accumulation of its stable break-down product 6-keto PGF 1α ( Fig. 7c,d ). However, our results also show that VEGF-A and VEGF-E promote much greater (>sixfold) 6-keto PGF 1α release from HUVEC than VEGF-E:PlGF-1 ( Fig. 7e ). Moreover, VEGF-A induced a tenfold increase in 6-keto PGF 1α release from PAER-2 cells while only eliciting a twofold release from PAER-1:R-2 cells ( Fig. 7f ). This finding suggests that VEGFR-2 homodimer activation is essential for strong VEGF-A-induced prostacyclin release and the presence of VEGFR-1 in PAER-2 cells negatively regulates prostacyclin release. To determine whether VEGFR 1−2 antagonizes the action of the VEGFR-2 homodimer receptor, we pre-treated HUVEC with VEGF-E:PlGF-1, stimulated them with either VEGF-A or VEGF-E and then assessed prostacyclin production ( Fig. 8a ). Interestingly, pre-incubation with VEGFR 1−2 significantly reduced the ability of VEGF-A and VEGF-E to stimulate prostacyclin release, whereas PlGF-1 had no inhibitory effect. These data suggest that the inhibitory signal for this response is exclusively via VEGFR 1−2 . 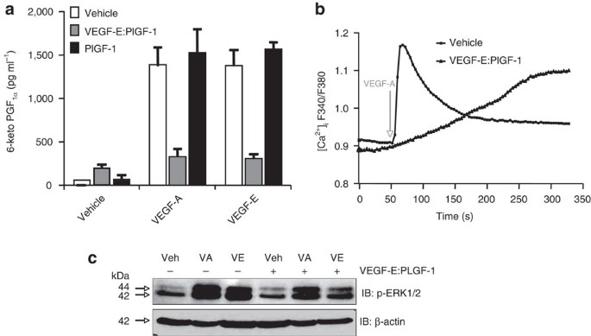Figure 8: VEGF-E:PlGF-1 inhibits VEGF-A-induced prostacyclin, calcium release and phosphorylation of ERK1/2 in endothelial cells. (a) HUVEC were rested overnight before preincubation with PlGF-1 or VEGF-E:PlGF-1 for 30 min and subsequent treatment with vehicle, VEGF-A and VEGF-E. Supernatants were collected and 6-keto PGF1αassessed by ELISA. (b) HUVEC were preincubated with vehicle or VEGF-E:PlGF-1 for 30 min, before addition of VEGF-A. Intracellular calcium release was assessed using Fura-2 AM. (c) HUVEC were preincubated with vehicle or VEGF-E:PlGF-1 for 30 min then stimulated with VEGF-A or VEGF-E for 15 min. radio immunoprecipitation assay lysates were subjected to SDS–PAGE and immunoblotting for phosphorylated ERK1/2. Results are expressed as mean (+s.e.m.) of at least three independent experiments. Figure 8: VEGF-E:PlGF-1 inhibits VEGF-A-induced prostacyclin, calcium release and phosphorylation of ERK1/2 in endothelial cells. ( a ) HUVEC were rested overnight before preincubation with PlGF-1 or VEGF-E:PlGF-1 for 30 min and subsequent treatment with vehicle, VEGF-A and VEGF-E. Supernatants were collected and 6-keto PGF 1α assessed by ELISA. ( b ) HUVEC were preincubated with vehicle or VEGF-E:PlGF-1 for 30 min, before addition of VEGF-A. Intracellular calcium release was assessed using Fura-2 AM. ( c ) HUVEC were preincubated with vehicle or VEGF-E:PlGF-1 for 30 min then stimulated with VEGF-A or VEGF-E for 15 min. radio immunoprecipitation assay lysates were subjected to SDS–PAGE and immunoblotting for phosphorylated ERK1/2. Results are expressed as mean (+s.e.m.) of at least three independent experiments. Full size image Activation of VEGFR-2 mobilizes calcium from intracellular stores [48] , and evidence derived from cell lines expressing specific VEGF receptor subtypes indicated that the heterodimer mediated induction of calcium release in a biphasic manner [32] . In our study, VEGF-A caused a rapid, but transient calcium release in HUVEC ( Fig. 8b ). Pre-incubation of HUVEC with VEGF-E:PlGF-1 before VEGF-A addition delayed calcium mobilization in response to VEGF-A, and was followed by a slower and more-sustained release of calcium ( Fig. 8b ). Finally, pre-incubation of HUVEC with VEGF-E:PLGF-1 inhibited phosphorylation of ERK1/2 by VEGF-A and VEGF-E ( Fig. 8c ). This study demonstrates the existence of preassembled VEGFR 1−2 heterodimer receptors in human primary endothelial cells and animal tissues, and identifies their physiological function. Recent computer modelling of VEGF receptor subunit dimerization predicted that heterodimerization would be inevitable when cells express both VEGFR-1 and VEGFR-2 subunits [34] . Furthermore, the model demonstrated that an excess of one VEGF receptor subunit would result in minimal homodimerization of the less abundant receptor subunit [34] . VEGFR-1 is known to be up to tenfold less abundant than VEGFR-2 on the endothelial cell surface [35] , [36] , implying that the majority of VEGFR-1 in endothelial cells exists in heterodimeric complexes with VEGFR-2. Our results show that VEGFR-1 predominantly modulates VEGF activity by forming heterodimers with VEGFR-2. To investigate the function of VEGFR 1−2 heterodimers in endothelial cells, we generated a selective ligand, comprising one monomer of VEGF-E (VEGFR-2-specific ligand) and one monomer of PlGF-1 (VEGFR-1-specific ligand). Use of PAEC expressing VEGFR-1, VEGFR-2, or both receptor subunits, confirmed the specificity of the ligand for the heterodimer receptor in binding and function. In addition, the FACS binding assay discounted the possibility that the respective monomers of VEGF-E:PlGF-1 would bind to homodimer receptors and thereby stoichiometrically block the binding of other VEGF ligands. The stimulation of murine lung capillary endothelial cells with VEGF-A was reported to increase the amount of VEGFR-1 associating with VEGFR-2 (ref. 19 ). In this study, we were unable to demonstrate an increase in receptor heterodimerization following ligand stimulation. This suggests that maximal heterodimerization occurs under basal conditions providing further evidence that the majority of VEGFR-1 subunits exist as preformed heterodimers with VEGFR-2 in HUVEC, as predicted by MacGabhann and Popel's computational model [34] . Although VEGF-A has a lower affinity for VEGFR-2 than VEGFR-1 (ref. 49 ), it is present in up to a tenfold excess of VEGFR-1. Therefore, VEGFR-1 subunits should exist as VEGFR 1−2 heterodimers and preferentially bind VEGF-A ahead of VEGFR-2 homodimers. We suggest that the presence of VEGFR-1-specific ligands such as PlGF and VEGF-B may be a mechanism for regulating VEGF receptor heterodimerization. Tyrosine phosphorylation of VEGFR-2, but not of VEGFR-1, could readily be detected after stimulation of VEGF-E:PlGF-1. Detecting VEGFR-1 phosphorylation consistently under native conditions is particularly difficult [41] , [42] . The fact that VEGF-E:PlGF-1 induces a significant increase in VEGFR-2 phosphorylation without binding to VEGFR-2 homodimers demonstrates that the VEGFR-2 subunit undergoes tyrosine phosphorylation when dimerized with a VEGFR-1 subunit. To assess the physiological effect of the VEGF-E:PlGF-1 heterodimer, we performed various in vitro assays with endothelial cells. The novel ligand mediated endothelial cell migration and VEGFR-1 promoter activity, and caused sustained in vitro tube formation to an extent comparable with VEGF-A and VEGF-E. These results suggest a role for VEGFR 1−2 in endothelial cell differentiation and maintenance. VEGFR 1−2 activation resulted in induction of ERK1/2 phosphorylation, but had no significant effect on cell proliferation, confirming previous findings that VEGF-A-induced proliferation is a VEGFR-2-mediated event [41] . VEGF-A regulates vessel tone via NO production, which is dependent on eNOS activation. In addition, eNOS phosphorylation and NO release are crucial for VEGF-mediated angiogenesis [16] , [50] , [51] . VEGF-A, PlGF-1 and VEGF-E:PlGF-1 caused significant relaxation of vessels precontracted with phenylephrine, whereas activation of the VEGFR-2 homodimer, using VEGF-E, did not increase vessel relaxation. This provides the first evidence that VEGF-A-induced vasorelaxation depends on the VEGFR-1 homodimer and/or the VEGFR 1−2 heterodimer, and does not require the VEGFR-2 homodimer. Endothelial VEGFR 1−2 activation also resulted in eNOS phosphorylation and NO release. VEGF-A-induced permeability requires the release of prostacyclin, an event initially attributed to VEGFR-2 homodimer action, because PlGF does not increase prostacyclin release [52] . However, use of VEGF-C and antisense knockdown of VEGF receptors led Neagoe and colleagues [33] to propose that VEGF-A-induced prostacyclin release was a VEGFR 1−2 -specific phenomenon. This study shows that VEGF-E, which exclusively activates the VEGFR-2 homodimer, induces ~15-fold increase in prostacyclin release from HUVEC. This indicates that VEGFR-2 homodimerization per se, can cause prostacyclin release from endothelial cells, whereas the magnitude of the VEGF-E:PlGF-1-induced increase in prostacyclin release was only threefold. This clearly demonstrates that although prostacyclin release can be mediated exclusively by the heterodimer receptor activation, it is predominantly a VEGFR-2 homodimer receptor function. Additionally, VEGF-A stimulation of PAER-2 induced a tenfold rise in prostacyclin release, whereas only a twofold release was apparent after VEGF-A stimulation of PAER-1:R-2. This finding suggests that VEGFR-1 negatively regulates prostacyclin release from endothelial cells. The convoluted approach taken by Neagoe and colleagues [33] to study VEGFR 1−2 heterodimerization further illustrates the benefit of this specific ligand. VEGF-A regulates its own bioactivity by a number of negative feedback systems; two examples are NO production [14] and sVEGFR-1 release [53] . In this study, we have shown that both of these functions are positively mediated by VEGFR 1−2 activation. Several groups have established that VEGFR-1 is a negative regulator of VEGFR-2-mediated endothelial and tumour cell proliferation [14] , [15] , [16] , [17] , [18] . Thus, we hypothesized that the overall function of VEGFR-1 forming heterodimeric receptors with VEGFR-2 may be to negatively regulate VEGFR-2 homodimer function in endothelial cells. Preincubation of HUVEC with VEGF-E:PlGF-1 abrogated VEGF-A and VEGF-E-mediated prostacyclin release, whereas preincubation with PlGF-1 had no effect. In addition, preincubation of cells with VEGF-E:PlGF-1 delayed the normally rapid and transient VEGF-A-mediated mobilization of intracellular cellular calcium and the eventual rise in calcium entry was much slower, but more sustained. Rapid increases in intracellular calcium generally equate to release from intracellular stores, whereas slower rises in intracellular calcium are due to influx from an extracellular source. The data suggest that VEGF-A alone, via VEGFR-2 can activate these intracellular stores. In contrast, VEGFR 1−2 activation elicits an inhibitory signal that delays this release. A subsequent dimension to receptor heterodimer function is the regulation of the activating ligand, be that VEGF-A or VEGF-A:PlGF. For the endogenous heterodimeric ligand (VEGF-A:PlGF) to be produced, there must be co-expression of both proteins in the same cell. A highly relevant publication has demonstrated that when this does occur, in a mouse tumour model, branching angiogenesis persists and monocyte migration into the tumours is enhanced [54] , thus showing a biological relevance of the heterodimer ligand and receptor. However, the contribution of VEGF-A and/or VEGF-A:PlGF to heterodimer receptor activation and cell function is likely to be regulated in a complicated spatial and temporal manner, which warrants future in-depth study in in vivo systems. In conclusion, data gathered using VEGF-E:PlGF-1 demonstrate that VEGFR 1−2 activation is functional in endothelial cells and that the heterodimer receptor serves as a negative regulator of the VEGFR-2 homodimer to regulate angiogenesis. This adds another layer of complexity to the regulation of VEGF-A function. It is possible that the low threshold homeostatic function of VEGF-A is achieved by the formation of the VEGFR 1−2 heterodimer, whereas pro-angiogenic and proliferative function is mediated by VEGFR-2 homodimers. We conclude that heterodimerization between VEGFR-1 and VEGFR-2 subunits, negatively regulates both the signalling and cell response of the VEGFR-2 homodimer. This may be important for angiogenesis and endothelial cell homeostasis. If validated in vivo , this concept would be a dramatic paradigm shift in the current understanding of VEGF receptor biology. Future studies should establish whether this mechanism is apparent in vivo and if heterodimerization is dysregulated in pathologies. Reagents and antibodies Growth factors and receptors were purchased from RELIATech (Brauschweig, Germany). Mouse anti-VEGFR-1 (Flt-11) was purchased from Sigma (Poole, UK). Mouse IgG, mouse anti-His-Tag, mouse anti-PY99 and rabbit anti-VEGFR-2 (C-1158) were obtained from Autogen Bioclear (Calne, UK). Rabbit polyclonal antiobodies against ERK1/2, phospho-ERK1/2 (tyr 402/thr 404), Akt, phospho-Akt (ser 463), endothelial nitric oxide synthase (eNOS), and phospho-eNOS (ser 1177) were obtained from NEB (Hitchin, UK). Mouse/goat anti-VEGFR-1 and VEGFR-2; and biotinylated goat anti-VEGFR-1, VEGFR-2 and phospho-tyrosine antibodies were purchased from R & D Systems (Abingdon, UK). Anti-PlGF [55] (clone 172) and anti-VEGF-E [39] were gifts from Dr Weich. MTT (3-(4,5-Dimethylthiazol–2-yl)-2,5-diphenyltetrazolium bromide) thiazolyl blue was purchased from Sigma-Aldrich (Poole, UK) and growth factor-reduced Matrigel obtained from Becton Dickinson (Oxford, UK). Sf21 insect cells, TC-100 and Sf 900 II medium were purchased from Invitrogen (Paisley, UK). Cell culture HUVEC were isolated and cultured as described previously [16] . Experiments were performed on third or fourth passage HUVEC. Human dermal microvascular endothelial cells (HMEC-1), immortalized by transformation with the SV-40 large T-antigen, were a gift from Dr E. Ades, Centre for Disease Control, Atlanta, USA. The PAEC expressing human VEGFR-1 (PAER-1) or VEGFR-2 (PAER-2) were maintained in medium supplemented with G418. PAER-1:R-2 were maintained in medium supplemented with zeocin. Sf 21 insect cells were expanded in spinner flasks in TC-100 medium supplemented with 5% FCS, maintained at 27 °C and infected with baculoviruses in serum-free Sf 900 II medium. Immunoprecipitation and western Blotting PAER-1:R-2, HMEC-1 and HUVEC lysed in radio immunoprecipitation assay buffer were immunoprecipiated using rabbit anti-VEGFR-2 (C-1158) or mouse anti-VEGFR-1. Membranes were incubated with mouse anti-PY99, mouse anti-VEGFR-1 (Flt-11), goat anti-VEGFR-1 or rabbit anti-VEGFR-2 (C-1158). After stimulations, HUVEC lysate was separated on SDS–PAGE and membranes probed with rabbit polyclonal antibodies, against signalling molecules, at 4 °C overnight. Supernatants from baculoviral infections were run on 15% gels and membranes probed with rabbit anti-PlGF-1 (1 in 100) or rabbit anti-VEGF-E (1 in 2,000). The same antibodies were used to detect PlGF and VEGF-E post purification. ELISA assay The ELISA for VEGFR 1−2 used anti-VEGFR-1 capture antibodies against either, the human or mouse protein and biotinylated anti-VEGFR-2 detection antibodies (R&D Systems). The ELISA for VEGF-E:PlGF-1 heterodimers used an anti-His-Tag capture antibody, an anti-VEGF-E detection and a goat anti-rabbit HRP conjugate. Phosphorylated VEGFR-2 was detected using a mouse anti-VEGFR-2 capture antibody and a biotinylated phospho-tyrosine detection antibody. The sVEGFR-1 concentration in cell supernatants was determined as described previously [12] . VEGFR-2 was measured in cell lysates using the VEGFR-2 ECD DuoSet ELISA (R&D Systems). 6-keto PGF 1α was measured in cell supernatants using the 6-keto PGF1α EIA kit (Biogenesis, Poole, UK). Expression and purification of recombinant VEGF-E:PlGF-1 The VEGF-E isoform used was isolated from the D1701 strain [39] and engineered to contain the VEGF-A-heparin-binding domain [40] . The cloning, expression and purification of 6xHis-tagged PlGF-1 and heparin-binding VEGF-E using a baculoviral system has already been described [40] , [55] . To produce VEGF-E:PlGF-1, Sf 21 insect cells were infected with baculoviruses encoding VEGF-E and PlGF-1. Clarified supernatant was then applied to a nickel chelating column (Ni-NTA; Qiagen, Crawley, UK) and bound proteins eluted with imidazole. The fractions containing PlGF-1 homodimers and VEGF-E:PlGF-1 heterodimers were identified by immunoblotting. VEGF-E-positive fractions were pooled, dialysed, loaded on a Heparin-Sepharose column (HiTrap Heparin; GE Healthcare, Amersham, UK), and eluted with a sodium chloride gradient [56] . After immunoblotting fractions positive for both proteins were pooled, dialysed against PBS and used for in vitro experiments. FACS analysis PAEC were incubated with VEGF-E:PlGF-1 (0.5 μg per 10 6 cells ml −1 ). Binding was detected using an anti-His-Tag and then a secondary FITC-conjugated anti-mouse. Flow cytometry was performed using a FACScan flow cytometer with CELLQuest software (Becton Dickinson, Oxford, UK) and the 488 nm argon laser. 15,000 cells were collected from each sample. Data were acquired in a list mode and three parameters checked; forward scatter, side scatter and one fluorescence channel (FL-1). siRNA transfection HUVEC were electroporated with siRNA duplexes to VEGFR-1 (sense, 5′-UGAUGGCCUUACACUGAAAtt-3′; antisense, 5′-UUUCAGUGUAAGGCCAUCAtt-3′), VEGFR-2 ( sense , 5′-GGAAAUCUCUUGCAAGCUAtt-3′; antisense, 5′-UAGCUUGCAAGAGAUUUCCtt-3′), neuropilin-1 (sense, 5′-GUAUACGGUUGCAAGAUAAtt-3′; antisense, 5′-UUAUCUUGCAACCGUAUACtt-3′), neuropilin-2 (sense, 5′-CCAGAAGAUUGUCCUCAACtt-3′; antisense, 5′-GUUGAGGACAAUCUUCUGGtt-3′) or universal control siRNA (Dharmacon) using the HUVEC kit II and AMAXA nucleofector (Lonza, Germany) [53] . Real-time PCR Total RNA of cultured cells was isolated using the total RNA Purification Kit (Norgen Biotek Corporation, Thorold, Canada) and 1 μg RNA was reverse-transcribed. Real-time PCR was performed for neuropilin-1 (sense 5′-CGCTCCCGCCTGAACTACCCT-3′; antisense, 5′-TGAGGTGCGGGTGGAAGTGCC-3′), neuropilin-2 (sense GGTGCGGGAAGCCAGCCAGGA; antisense GCCCCCAGGAGGACGCCCAGT) and β-actin [57] using SYBR green and SensiMix (dT) DNA Kit (Quantace, London, UK) on a RotorGene 3000 (Corbett Research, Sydney, Australia). For each run, a standard curve was prepared alongside the sample complementary DNAs. Relative neuropilin-1/2 mRNA expression was calculated from the ΔCt values following normalization to β-actin levels. PCR products were run on 2% agarose gel to verify product size (neuropilin-1: 521 bp; neuropilin-2: 447 bp) and purity. Immunofluorescence imaging HUVEC were stimulated with growth factors and fixed with 4% (w/v) paraformaldehyde. To determine cell surface VEGFR-1 and VEGFR-2 expression after stimulations, fixed cells were incubated with primary antibodies goat-anti-VEGFR-1 (R&D Systems; 1 in 10), rabbit-anti-VEGFR-2 (Cell Signaling; 1 in 20), respectively, then FITC-labelled anti-goat (Sigma; 1 in 200) and TRITC-labelled anti-rabbit secondary antibodies (Cell Signaling; 1 in 200). To determine VEGF-E trafficking in HUVECs after stimulation, cells permeabilized with ice-cold methanol were incubated with rabbit-anti-VEGF-E antibody (ReliaTECH) then TRITC-labelled anti-rabbit secondary antibody (Sigma). To determine VEGFR-1 and VEGFR-2 co-localization, permeabilized HUVEC were incubated with both goat anti-VEGFR-1 and rabbit anti-VEGFR-2 primary antibodies and detected with FITC-labelled anti-goat and TRITC-labelled anti-rabbit secondary antibodies. Cells were counterstained with DAPI, and viewed using a Zeiss LSM 510 confocal scanning microscope (Carl Zeiss, Jena, Germany). Images were analysed using LSM 510 software (version 2.3; Carl Zeiss). In vitro migration Chemotaxis experiments with HUVEC, HMEC, PAEC and PBMC were performed in a modified Boyden chamber [16] . Cells migrated towards growth factor gradients for 6 h through 8 μm PVP-free membranes. Membranes were then fixed in methanol, stained with Diff-Quik (Harleco, USA) and cell migration quantified by counting 8–10 fields of view at X10 magnification. VEGFR-1 promoter reporter assay PAER-1 and PAER-1:R-2 were transfected with a luciferase reporter construct containing ~1.3 kb. fragment of the human VEGFR-1 promoter using Exgen 500 (Fermentas, York, UK) before incubation with VEGF-A or VEGF-E:PlGF-1 and promoter activity determined with a luminometer. Coagulation assay Confluent HUVEC monolayers were stimulated with growth factors for 6 h, and a coagulation assay was performed and clotting times converted to tissue factor equivalents [58] . In vitro tube formation assay Formation of capillary-like structures on growth-factor reduced Matrigel was determined, as previously described [16] . MTT assay Confluent HUVEC were rested overnight in medium containing 5% FCS, then stimulated with growth factors for 96 h. MTT (5 mg ml −1 ) was added and the cells incubated in the dark at 37 °C for 4 h. MTT was aspirated and reconstituted in dimethylsulphoxide. Optical density values were measured at 540 and 690 nm. Myography All experiments were performed according to the Animals Scientific Procedures Act 1986 (U.K. Home Office) [59] . Briefly, adult male Wistar rats (250–400 g; Charles River, Margate, UK) were killed by cervical dislocation. The thoracic aorta was dissected free, cleaned and ~5 mm length sections mounted in a multi-myograph system (610M; Danish Myo Technology, Aarhus, Denmark) in Krebs buffer bubbled with 5% CO2/95% O2 at 37 °C. A baseline tension of 14.7 mN was gradually applied over 10 min and vessels were allowed to equilibrate for a further 30 min before challenge with 80 mM KCl to assess viability. Phenylephrine was used to precontract vessels to ~80% maximum contraction (EC 80 ; ~0.2 μM) for each individual aortic ring. Following precontraction, cumulative concentration response curves to VEGF ligands (0.01–1 nM) were performed in separate vessel segments. Drugs were washed out and concentration response curves were repeated in the presence (20 min preincubation and presence throughout concentration response curve) of the nitric oxide synthase inhibitor N ω -Nitro- L -arginine methyl ester ( L -NAME; 200 μM) and the cyclooxygenase inhibitor indomethacin (10 μM). The data from force transducers were processed by a MacLab/4e analog–digital converter and displayed through Chart software, version 3.4.3 (AD Instruments, Sussex, UK). Analysis of NO release Confluent HUVEC were incubated with growth factors in medium containing 0.2%. BSA, for 1 h at 37 °C. Total NO in the culture medium was assayed as nitrite, the stable breakdown product of NO, using a Sievers NO chemiluminescence analyzer (Analytix, Sunderland, UK). Calcium imaging HUVEC were grown to 90% confluency on gelatin-coated coverslips, and loaded with the calcium sensitive dye, Fura-2 AM (Molecular Probes, UK), for 30 min. After rinsing, growth factors were added and the change in calcium influx was dynamically assayed over a 2-min period. Statistical analysis All data are expressed as mean±s.e.m. Statistical comparisons were performed using one-way ANOVA followed by the Student—Newman–Keuls test as appropriate. Statistical significance was set at a value of P <0.05. How to cite this article: Cudmore, M.J. et al . The role of heterodimerization between VEGFR-1 and VEGFR-2 in the regulation of endothelial cell homeostasis. Nat. Commun. 3:972 doi: 10.1038/ncomms1977 (2012).